Blockade of TLR3 protects mice from lethal radiation-induced gastrointestinal syndrome High-dose ionizing radiation induces severe DNA damage in the epithelial stem cells in small intestinal crypts and causes gastrointestinal syndrome (GIS). Although the tumour suppressor p53 is a primary factor inducing death of crypt cells with DNA damage, its essential role in maintaining genome stability means inhibiting p53 to prevent GIS is not a viable strategy. Here we show that the innate immune receptor Toll-like receptor 3 (TLR3) is critical for the pathogenesis of GIS. Tlr3 −/− mice show substantial resistance to GIS owing to significantly reduced radiation-induced crypt cell death. Despite showing reduced crypt cell death, p53-dependent crypt cell death is not impaired in Tlr3 −/− mice. p53-dependent crypt cell death causes leakage of cellular RNA, which induces extensive cell death via TLR3. An inhibitor of TLR3–RNA binding ameliorates GIS by reducing crypt cell death. Thus, we propose blocking TLR3 activation as a novel approach to treat GIS. Acute radiation syndrome is an acute illness that occurs upon exposure to high amounts of ionizing radiation. In acute radiation syndrome, various symptoms appear according to the radiation sensitivity of each organ [1] , [2] , [3] . In humans, after whole-body exposure to a 1.5-Gy total dose, hematopoietic stem cells, one of the most radio-sensitive cell types in the body, are severely affected. Exposure leads to a haemorrhagic tendency and immunological deterioration owing to insufficient supply of platelets and leukocytes, respectively (hematopoietic syndrome; HPS) [1] , [2] , [3] . To prevent death from HPS, infection control and hematopoietic stem cell transplantation are performed as a medical treatment. Above 5 Gy, exposed persons suffer from severe intestinal injury, which causes subacute death with diarrhea, malabsorption and bacterial enteritis (gastrointestinal syndrome; GIS) [1] , [2] , [3] . Unfortunately, in contrast to HPS, no effective treatments for GIS have been developed to date. It has been generally accepted that GIS results from death of the epithelial stem cells in the crypts of Lieberkühn [2] , [3] . When ionizing radiation damages host DNA, the tumour suppressor gene p53 induces cell cycle arrest for DNA repair [4] . If the DNA damage turns out to be irreparable, p53 initiates programmed cell death. p53-mediated cell death in crypt epithelial cells has been implicated as the direct trigger of GIS [5] . In contrast, other groups have proposed that GIS is regulated by cell death of endothelial cells within the intestinal microvascular network via ceramide generation on the external plasma membrane [6] . However, this concept remains controversial [7] . Moreover, a recent report indicated that survival from GIS is not determined by the amount of cell death of endothelial cells [8] . Although drugs that block p53-mediated cell death of crypt epithelial cells are expected to prevent GIS, therapeutic application of p53 inhibitors is problematic because of the adverse effect on DNA repair. Innate immunity recognizes invasion of microorganisms and serves as a first line of defence against infection [9] , [10] . The Toll-like receptor (TLR) family is one of the best-characterized families of innate immune receptors, which recognize microbial components and induce the innate immune response against pathogens [9] , [10] . In addition, previous studies have also supported the protective function of TLRs against radiation damage to the gastrointenstinal (GI) tract. Stimulation of TLR2 with probiotic lactobacilli and of TLR4 with lipopolysaccharide before irradiation results in radioprotective effects on the mouse intestine through a mechanism dependent on cyclo-oxygenase-2 (refs 11 , 12 ). Pretreatment with a polypeptide drug derived from Salmonella flagellin, which is a ligand for TLR5, protected both mice and monkeys from GIS [13] . A recent study showed that a synthetic TLR9 agonist mitigates GIS in mice, possibly through activating the regenerative functions of intestinal macrophages [14] . Thus, manipulation of TLR functions is gaining attention as a potent prophylactic tool against GIS. To analyse the role of TLR3 in GIS, we examine the effects of the TLR3 ligand polyinosinic-polycytidylic acid (poly I:C) and show that poly I:C treatment aggravates, rather than ameliorates, GIS in a TLR3-dependent manner. Intriguingly, regardless of poly I:C treatment, Tlr3 −/− mice show marked resistance to GIS owing to significant reduction of radiation-induced crypt cell death. p53-dependent crypt cell death causes leakage of cellular RNA, which induces extensive cell death via TLR3. We demonstrate that a TLR3/double-stranded (ds) RNA complex inhibitor effectively ameliorates crypt cell death and GIS. Thus, our findings provide a new framework to understand the pathogenesis of GIS and suggest blockade of TLR3 as a new therapeutic strategy for the treatment of GIS. TLR3 is an exacerbating factor for radiation-induced GIS To investigate the influence of TLR3 activation on GIS, we treated Tlr3 +/+ and Tlr3 −/− mice on a BALB/c background with the synthetic TLR3 ligand poly I:C (ref. 15 ) before total body γ-irradiation (TBI). As BALB/c mice are known to be sensitive to irradiation, 10-Gy TBI was performed to examine radiation susceptibility [16] . Poly I:C treatment did not protect mice and significantly increased the susceptibility of Tlr3 +/+ mice to TBI ( Fig. 1a ). We also examined diarrhea and body weight loss after irradiation, which are the major symptoms of GIS [2] , [3] . The severity of diarrhea in non-treated Tlr3 +/+ mice got progressively worse from day 3 after TBI, while poly I:C-treated Tlr3 +/+ mice showed more severe symptoms from day 1 ( Fig. 1b ). In addition, poly I:C treatment significantly promoted body weight loss in Tlr3 +/+ mice ( Fig. 1c ). Contrary to Tlr3 +/+ mice, poly I:C treatment had no effects on the severity of diarrhea and body weight loss following TBI in Tlr3 −/− mice. Thus, poly I:C stimulation of TLR3 exacerbates radiation-induced GIS. Intriguingly, Tlr3 −/− mice showed significantly milder symptoms of GIS, including mortality, diarrhea and body weight loss, compared with Tlr3 +/+ mice, regardless of poly I:C treatment. We then examined the susceptibility of mice deficient in other TLR family members to radiation-induced GIS. However, unlike Tlr3 −/− mice, mice deficient in other TLRs showed no changes in survival, diarrhea and weight loss following TBI when compared with wild-type mice ( Supplementary Fig. 1a–c ). We next examined HPS in Tlr3 −/− mice; however, there were no differences in bone marrow (BM) suppression and leucopenia between Tlr3 +/+ and Tlr3 −/− mice after TBI ( Fig. 1d–f ). Thus, TLR3 is specifically activated after TBI and contributes to exacerbation of GIS. 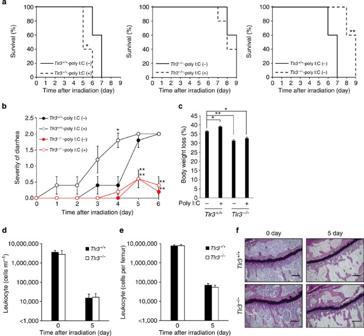Figure 1: Activation of TLR3 exacerbates radiation-induced GIS. (a) Kaplan–Meier survival analyses ofTlr3+/+andTlr3−/−mice after TBI with or without poly I:C pretreatment.n=5; *P<0.05; **P<0.01 (log-rank test). (b) Severity of diarrhea ofTlr3+/+andTlr3−/−mice after TBI with or without poly I:C pretreatment.n=5; results are means±s.e.m. *P<0.05; **P<0.01 (unpaired two-tailed Student’st-test). (c) Body weight loss ofTlr3+/+andTlr3−/−mice on day 5 after TBI with or without poly I:C pretreatment.n=5; results are means±s.e.m. *P<0.05; **P<0.01 (unpaired two-tailed Student’st-test). (d) The numbers of blood leukocytes and (e) BM leukocytes ofTlr3+/+andTlr3−/−mice 0 and 5 days after TBI.n=3. results are means±s.e.m. (f) H&E staining of tibiae at days 0 and 5. Scale bar, 200 μm. Results are representative of three independent experiments. Figure 1: Activation of TLR3 exacerbates radiation-induced GIS. ( a ) Kaplan–Meier survival analyses of Tlr3 +/+ and Tlr3 −/− mice after TBI with or without poly I:C pretreatment. n =5; * P <0.05; ** P <0.01 (log-rank test). ( b ) Severity of diarrhea of Tlr3 +/+ and Tlr3 −/− mice after TBI with or without poly I:C pretreatment. n =5; results are means±s.e.m. * P <0.05; ** P <0.01 (unpaired two-tailed Student’s t -test). ( c ) Body weight loss of Tlr3 +/+ and Tlr3 −/− mice on day 5 after TBI with or without poly I:C pretreatment. n =5; results are means±s.e.m. * P <0.05; ** P <0.01 (unpaired two-tailed Student’s t -test). ( d ) The numbers of blood leukocytes and ( e ) BM leukocytes of Tlr3 +/+ and Tlr3 −/− mice 0 and 5 days after TBI. n =3. results are means±s.e.m. ( f ) H&E staining of tibiae at days 0 and 5. Scale bar, 200 μm. Results are representative of three independent experiments. Full size image TLR3 mediates crypt cell death in radiation-induced GIS To preclude a possible influence of HPS, we performed isologous BM transplantation (BMT) in Tlr3 +/+ and Tlr3 −/− mice immediately after TBI. Whereas TBI was lethal for Tlr3 +/+ BMT mice, all Tlr3 −/− BMT mice survived at the same dose ( Fig. 2a ), implying that irradiated Tlr3 −/− mice died from HPS. Compared with Tlr3 +/+ BMT mice, both diarrhea symptoms and body weight loss were significantly milder in Tlr3 −/− BMT mice ( Fig. 2b,c ). Thus, GIS was attenuated in Tlr3 −/− mice. We also prepared Tlr3 +/+ mice that received BM cells from Tlr3 −/− mice and Tlr3 −/− mice that received BM cells from Tlr3 +/+ mice. As a result, regardless of donor cells, GIS was attenuated in Tlr3 −/− recipients, suggesting that TLR3 on non-BM cells, but not on BM cells, significantly contributes to the pathogenesis of GIS ( Supplementary Fig. 2a–c ). We next performed TUNEL assays to examine cell death of crypt epithelial cells in the small intestine. As shown in Fig. 2d and Supplementary Fig. 3 , the number of TUNEL-positive cells per crypt in Tlr3 −/− mice was much lower than that in Tlr3 +/+ mice 6 h post TBI. Thus, TLR3 was involved in crypt cell death after irradiation. Whereas crypt microcolonies, a surrogate indicator of crypt regeneration [17] , were rarely observed in the small intestine of Tlr3 +/+ mice 3 days after TBI, Tlr3 −/− mice had significantly higher numbers of crypt microcolonies ( Fig. 2e ). We further examined the proliferation of crypt cells on day 3 after TBI. Although BrdU-labelled cells were scarcely detected in the crypts of Tlr3 +/+ mice, the numbers of BrdU-labelled crypt cells in Tlr3 −/− mice were vastly greater ( Fig. 2f ). We next compared the histological manifestations of GIS in the small intestine between Tlr3 +/+ and Tlr3 −/− mice after TBI. Tlr3 −/− mice showed a normal small intestine structure comparable to that in Tlr3 +/+ mice before TBI ( Fig. 2g ), suggesting that TLR3 is not involved in organogenesis of the small intestine. At day 5, evidence of villous destruction, such as blunting, fusion and epithelial denudation, was observed in the small intestine of Tlr3 +/+ mice, whereas the villus structure of the small intestine was still preserved in Tlr3 −/− mice ( Fig. 2g ). Although we examined cell death in the villous epithelium, we hardly observed any increase in the number of TUNEL-positive cells in either Tlr3 +/+ or Tlr3 −/− mice 6 h and 3 days after TBI ( Supplementary Fig. 4 ). Furthermore, there was scarcely any accumulation of inflammatory cells in the small intestinal villi of Tlr3 +/+ and Tlr3 −/− mice 6 h and 3 days after TBI ( Supplementary Fig. 4 ). Thus, neither radiation-induced epithelial cell death nor inflammation affected villous integrity. Taken together, these findings indicate that radiation-induced crypt cell death was milder in Tlr3 −/− mice than in Tlr3 +/+ mice, leading to the presence of regenerating crypts at day 3, the subsequent normal re-epithelization of small intestinal villi at day 5, and prevention of GIS-induced death. 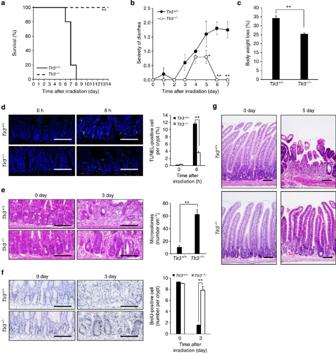Figure 2:Tlr3−/−mice avoid GIS because of reduction in radiation-induced crypt cell death. (a) Kaplan–Meier survival analysis ofTlr3+/+andTlr3−/−mice treated with TBI and isologous BMT.n=5; **P<0.01 (log-rank test). (b) Severity of diarrhea ofTlr3+/+andTlr3−/−mice.n=5; results are means±s.e.m. *P<0.05; **P<0.01 (unpaired two-tailed Student’st-test). (c) Body weight loss ofTlr3+/+andTlr3−/−mice at day 5.n=5; results are means±s.e.m. **P<0.01 (unpaired two-tailed Student’st-test). (d) TUNEL-staining of the small intestines ofTlr3+/+andTlr3−/−mice at 0 and 6 h. TUNEL-stained epithelium shows green fluorescence. Nuclei were stained with DAPI (blue). Scale bar, 100 μm. The right-hand panel shows numbers of TUNEL-positive cells.n=4; results are means±s.e.m. **P<0.01 (unpaired two-tailed Student’st-test). (e) H&E staining of the small intestinal crypts ofTlr3+/+andTlr3−/−mice at days 0 and 3. Scale bar, 100 μm. Asterisks denote microcolonies. Right panel shows the numbers of microcolonies.n=3; results are means±s.e.m. **P<0.01 (unpaired two-tailed Student’st-test). (f) Immunohistochemical detection of BrdU in small intestinal crypts ofTlr3+/+andTlr3−/−mice at days 0 and 3. Scale bar, 100 μm. The right-hand panel shows the numbers of BrdU-incorporating cells.n=3; results are means±s.e.m. **P<0.01 (unpaired two-tailed Student’st-test). (g) H&E staining ofTlr3+/+andTlr3−/−small intestines at days 0 and 5. Scale bar, 100 μm. Results are representative of three independent experiments. Figure 2: Tlr3 −/− mice avoid GIS because of reduction in radiation-induced crypt cell death. ( a ) Kaplan–Meier survival analysis of Tlr3 +/+ and Tlr3 −/− mice treated with TBI and isologous BMT. n =5; ** P <0.01 (log-rank test). ( b ) Severity of diarrhea of Tlr3 +/+ and Tlr3 −/− mice. n =5; results are means±s.e.m. * P <0.05; ** P <0.01 (unpaired two-tailed Student’s t -test). ( c ) Body weight loss of Tlr3 +/+ and Tlr3 −/− mice at day 5. n =5; results are means±s.e.m. ** P <0.01 (unpaired two-tailed Student’s t -test). ( d ) TUNEL-staining of the small intestines of Tlr3 +/+ and Tlr3 −/− mice at 0 and 6 h. TUNEL-stained epithelium shows green fluorescence. Nuclei were stained with DAPI (blue). Scale bar, 100 μm. The right-hand panel shows numbers of TUNEL-positive cells. n =4; results are means±s.e.m. ** P <0.01 (unpaired two-tailed Student’s t -test). ( e ) H&E staining of the small intestinal crypts of Tlr3 +/+ and Tlr3 −/− mice at days 0 and 3. Scale bar, 100 μm. Asterisks denote microcolonies. Right panel shows the numbers of microcolonies. n =3; results are means±s.e.m. ** P <0.01 (unpaired two-tailed Student’s t -test). ( f ) Immunohistochemical detection of BrdU in small intestinal crypts of Tlr3 +/+ and Tlr3 −/− mice at days 0 and 3. Scale bar, 100 μm. The right-hand panel shows the numbers of BrdU-incorporating cells. n =3; results are means±s.e.m. ** P <0.01 (unpaired two-tailed Student’s t -test). ( g ) H&E staining of Tlr3 +/+ and Tlr3 −/− small intestines at days 0 and 5. Scale bar, 100 μm. Results are representative of three independent experiments. Full size image TLR3 directly induces cell death in small intestinal crypts As there was a difference in the degree of crypt cell death after TBI between Tlr3 +/+ and Tlr3 −/− mice, we examined whether TLR3 is directly involved in this event. As shown by Fig. 3a and Supplementary Fig. 5 , crypt epithelial cells expressed high levels of Tlr3 mRNA. We therefore examined how poly I:C affects crypt cells using the in vitro crypt culture method [18] . We cultured small intestinal crypts from Tlr3 +/+ and Tlr3 −/− mice in a Matrigel-based culture system for 6 days ( Fig. 3b ). Both Tlr3 +/+ and Tlr3 −/− crypts formed crypt–villus organoids in a similar fashion, in which crypt domains surrounded the central lumen lined by a villus-like epithelium and underwent continuous budding events. Poly I:C administration led to a disappearance of crypt domains in Tlr3 +/+ organoids. In contrast, the structures of crypt–villus organoids were preserved in Tlr3 −/− organoids regardless of poly I:C stimulation. We also assessed the cell viability of Tlr3 +/+ and Tlr3 −/− organoids by MTT assay ( Fig. 3c ). While the cell viability of Tlr3 +/+ organoids was dramatically decreased after poly I:C treatment, the viability did not change in Tlr3 −/− organoids. Moreover, whole-mount analysis demonstrated that poly I:C stimulation increased the numbers of TUNEL-positive cells in the crypt domains of Tlr3 +/+ but not Tlr3 −/− organoids ( Fig. 3d ). We further examined the effect of poly I:C on the small intestinal crypt in vivo. Intraperitoneal injection of poly I:C significantly induced the appearance of TUNEL-positive crypt cells in Tlr3 +/+ mice, but not in Tlr3 −/− mice ( Fig. 3e ). Thus, ligand stimulation of TLR3 can directly induce extensive cell death in the crypt epithelium. 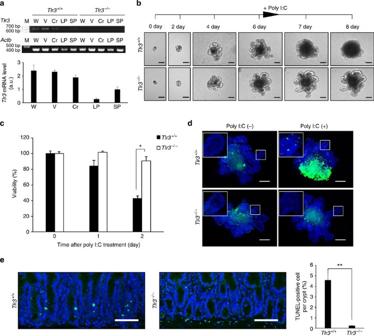Figure 3: Ligand stimulation of TLR3 directly induces cell death in small intestinal crypts. (a) RT-PCR (top) and quantitative real-time PCR (bottom) ofTlr3mRNA in the small intestines ofTlr3+/+andTlr3−/−mice. Cr, crypt; LP, lamina propria; M, size marker; SP, spleen; V, villi; W, whole intestine.n=3; results are means±s.e.m. (b) Representative images ofTlr3+/+andTlr3−/−organoids. Crypts were incubated with poly I:C after day 6 of culture. Scale bar, 100 μm. (c) Viability ofTlr3+/+andTlr3−/−organoids after poly I:C treatment.n=4; results are means±s.e.m. *P<0.05 (unpaired two-tailed Student’st-test). (d) TUNEL-staining ofTlr3+/+andTlr3−/−organoids at 1 day after poly I:C treatment. TUNEL-stained epithelium shows green fluorescence. Nuclei were stained with DAPI (blue). Insets show higher magnification of the crypt-like domain. Scale bar, 100 μm. (e) TUNEL-staining of the small intestinal crypts ofTlr3+/+andTlr3−/−mice 6 h after poly I:C injection. TUNEL-stained epithelium shows green fluorescence. Nuclei were stained with DAPI (blue). Scale bar, 100 μm. The right-hand panel shows numbers of TUNEL-positive cells.n=3; results are means±s.e.m. **P<0.01 (unpaired two-tailed Student’st-test). Results are representative of three independent experiments. Figure 3: Ligand stimulation of TLR3 directly induces cell death in small intestinal crypts. ( a ) RT-PCR (top) and quantitative real-time PCR (bottom) of Tlr3 mRNA in the small intestines of Tlr3 +/+ and Tlr3 −/− mice. Cr, crypt; LP, lamina propria; M, size marker; SP, spleen; V, villi; W, whole intestine. n =3; results are means±s.e.m. ( b ) Representative images of Tlr3 +/+ and Tlr3 −/− organoids. Crypts were incubated with poly I:C after day 6 of culture. Scale bar, 100 μm. ( c ) Viability of Tlr3 +/+ and Tlr3 −/− organoids after poly I:C treatment. n =4; results are means±s.e.m. * P <0.05 (unpaired two-tailed Student’s t -test). ( d ) TUNEL-staining of Tlr3 +/+ and Tlr3 −/− organoids at 1 day after poly I:C treatment. TUNEL-stained epithelium shows green fluorescence. Nuclei were stained with DAPI (blue). Insets show higher magnification of the crypt-like domain. Scale bar, 100 μm. ( e ) TUNEL-staining of the small intestinal crypts of Tlr3 +/+ and Tlr3 −/− mice 6 h after poly I:C injection. TUNEL-stained epithelium shows green fluorescence. Nuclei were stained with DAPI (blue). Scale bar, 100 μm. The right-hand panel shows numbers of TUNEL-positive cells. n =3; results are means±s.e.m. ** P <0.01 (unpaired two-tailed Student’s t -test). Results are representative of three independent experiments. Full size image TLR3 induces crypt cell death post TBI via TRIF–RIP1 pathway TLRs are composed of an ectodomain, a transmembrane domain and a cytosolic signalling domain known as the Toll-interleukin 1 receptor homology (TIR) domain [9] . TLR recognizes the ligand through its ectodomain, which induces homotypic binding of TIR domains in the receptors with those in adaptor molecules for signal transduction. Unlike other TLR family members, TLR3 does not utilize the common adaptor myeloid differentiation factor 88 (MyD88) [19] , [20] . Instead, TLR3 recruits another adaptor molecule TIR-domain-containing adapter-inducing interferon-β (TRIF) (also known as TIR-containing adaptor molecule-1; TICAM-1), which induces the activation of interferon regulatory factor 3 (IRF3) for the transcription of type I interferon (IFN) genes [20] . We investigated the role of TRIF in GIS. Similar to Tlr3 −/− mice, Trif −/− mice survived significantly longer after 10-Gy TBI than did Trif +/+ mice ( Supplementary Fig. 6a ). Compared with Trif +/+ mice, both diarrhea symptoms and body weight loss were significantly milder in Trif −/− mice ( Supplementary Fig. 6b,c ). Consistent with the survival and symptoms, crypt cell death and crypt survival were milder in Trif −/− mice than in Trif +/+ mice ( Fig. 4a,b ). Thus, Trif −/− mice showed a similar phenotype to that of Tlr3 −/− mice after 10-Gy TBI. We further investigated the contributions of IRF3 and type I IFN receptor (IFNAR) to GIS using Irf3 −/− and Ifnar −/− mice. Interestingly, there were no significant differences in survival, diarrhea, body weight loss and crypt damage between Irf3 +/+ and Irf3 −/− mice ( Fig. 4a,b and Supplementary Fig. 7a–c ). Furthermore, Ifnar −/− mice showed no difference from Ifnar +/+ mice in terms of survival, symptoms and crypt damage ( Fig. 4a,b and Supplementary Fig. 8a–c ). Thus, IRF3 and type I IFN are not involved in the pathogenesis of GIS. Although the N-terminal region of TRIF is essential for TRIF-mediated IRF3 activation, the C-terminal region has been reported to be crucial for NF-κB activation and cell death. Receptor-interacting protein 1 (RIP1), a kinase harbouring a death domain, associates with TRIF via the RIP homotypic interaction motif domain in the C-terminal region and transmits signals for NF-κB activation and cell death [21] , [22] . To examine the involvement of RIP1 in GIS after TBI, we treated mice with necrostatin-1 (Nec-1), an RIP1-specific allosteric inhibitor [23] . Nec-1 treatment resulted in an improvement in survival and diarrhea symptoms, although there were no significant effects on the amount of body weight loss ( Supplementary Fig. 9a–c ). Moreover, Nec-1 treatment significantly reduced the number of TUNEL-positive crypt cells 6 h and increased the number of microcolonies 3 days after TBI ( Fig. 4c,d ). Taken together, these findings suggest that TLR3 mediates radiation-induced crypt cell death through the TRIF–RIP1 pathway. 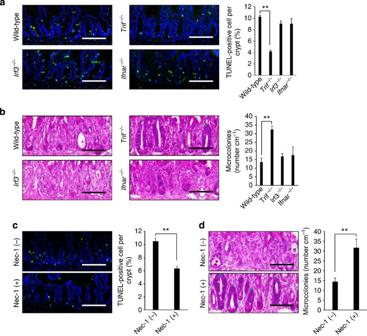Figure 4: TLR3 mediates radiation-induced crypt cell death through the TRIF–RIP1 pathway. (a) TUNEL-staining of the small intestinal crypts ofTrif−/−,Irf3−/−andIfnar−/−mice 6 h after TBI and isologous BMT. TUNEL-stained epithelium shows green fluorescence. Nuclei were stained with DAPI (blue). Scale bar, 100 μm. The right-hand panel shows numbers of TUNEL-positive cells.n=3–4; results are means±s.e.m. **P<0.01 (unpaired two-tailed Student’st-test). (b) H&E staining of the small intestinal crypts ofTrif−/−,Irf3−/−andIfnar−/−mice at day 3. Scale bar, 100 μm. Asterisks denote microcolonies. The right-hand panel shows the numbers of microcolonies.n=3–5; results are means±s.e.m. **P<0.01 (unpaired two-tailed Student’st-test). (c) TUNEL-staining of the small intestinal crypts of non-treated and Nec-1-treated mice 6 h after TBI and isologous BMT. TUNEL-stained epithelium shows green fluorescence. Nuclei were stained with DAPI (blue). Scale bar, 100 μm. The right-hand panel shows numbers of TUNEL-positive cells.n=5; results are means±s.e.m. **P<0.01 (unpaired two-tailed Student’st-test). (d) H&E staining of the small intestinal crypts of non-treated and Nec-1-treated mice at day 3. Scale bar, 100 μm. Asterisks denote microcolonies. Right panel shows the numbers of microcolonies.n=5; results are means±s.e.m. **P<0.01 (unpaired two-tailed Student’st-test). Results are representative of three independent experiments. Figure 4: TLR3 mediates radiation-induced crypt cell death through the TRIF–RIP1 pathway. ( a ) TUNEL-staining of the small intestinal crypts of Trif −/− , Irf3 − / − and Ifnar − / − mice 6 h after TBI and isologous BMT. TUNEL-stained epithelium shows green fluorescence. Nuclei were stained with DAPI (blue). Scale bar, 100 μm. The right-hand panel shows numbers of TUNEL-positive cells. n =3–4; results are means±s.e.m. ** P <0.01 (unpaired two-tailed Student’s t -test). ( b ) H&E staining of the small intestinal crypts of Trif −/− , Irf3 − / − and Ifnar − / − mice at day 3. Scale bar, 100 μm. Asterisks denote microcolonies. The right-hand panel shows the numbers of microcolonies. n =3–5; results are means±s.e.m. ** P <0.01 (unpaired two-tailed Student’s t -test). ( c ) TUNEL-staining of the small intestinal crypts of non-treated and Nec-1-treated mice 6 h after TBI and isologous BMT. TUNEL-stained epithelium shows green fluorescence. Nuclei were stained with DAPI (blue). Scale bar, 100 μm. The right-hand panel shows numbers of TUNEL-positive cells. n =5; results are means±s.e.m. ** P <0.01 (unpaired two-tailed Student’s t -test). ( d ) H&E staining of the small intestinal crypts of non-treated and Nec-1-treated mice at day 3. Scale bar, 100 μm. Asterisks denote microcolonies. Right panel shows the numbers of microcolonies. n =5; results are means±s.e.m. ** P <0.01 (unpaired two-tailed Student’s t -test). Results are representative of three independent experiments. Full size image It has been suggested that TLR3 induces two different types of cell death, apoptosis and necroptosis, in a cell type-specific manner [24] . Apoptosis occurs through activation of members of the caspase family in response to ligand stimulation of death receptors and to intracellular damage [24] . In TLR3-mediated apoptosis, TRIF binding with RIP1 induces downstream signalling through Fas-associated protein with death domain (FADD) and caspase-8, which subsequently cleaves the effector caspase-3 to execute apoptosis [25] , [26] . In contrast, necroptosis is a programmed form of necrotic cell death induced by death domain receptors activated by their ligands, under conditions when caspase function is absent or inhibited [24] . We observed an increase in the number of active caspase-3-positive cells in the crypts of Tlr3 +/+ mice after TBI and poly I:C injection ( Supplementary Fig. 10 ). In Tlr3 −/− mice, the number of active caspase-3-positive crypt cells after TBI and poly I:C injection was significantly suppressed. Thus, apoptosis is the type of crypt cell death induced by the TLR3 pathway after TBI. TLR3-mediated crypt cell death after TBI depends on p53 p53 has been implicated as a primary causal factor in radiation-induced crypt cell death [5] . Ionizing radiation induces the phosphorylation of the p53 protein, which prevents its ubiquitination and subsequent proteasomal degradation [5] . p53 phosphorylation results in the nuclear accumulation of transcriptionally active p53, leading to the induction of pro-apoptotic genes such as Bcl-2-associated X protein (Bax) and p53-upregulated modulator of apoptosis (PUMA). In fact, the numbers of TUNEL-positive crypt cells as well as induction of Bax and Puma mRNA were almost completely diminished in p53 −/− mice 6 h post TBI ( Fig. 5a,b ). Hence, crypt cell death 6 h after TBI is p53-dependent. Interestingly, TUNEL-positive crypt cells were still detected in Tlr3 −/− mice 6 h post TBI ( Fig. 2d ). Accumulation of p53 protein in the crypt cells and upregulation of Bax and Puma mRNA in the small intestines of Tlr3 +/+ and Tlr3 −/− mice were significantly induced to a similar extent 6 h after TBI ( Fig. 5c,d ). Thus, p53-mediated cell death signalling after TBI was not impaired in Tlr3 −/− mice. According to a recent report, TLR3 induction is regulated by p53 in several cancer cell lines [27] . However, there was no significant difference in Tlr3 mRNA expression in the small intestine between p53 +/+ and p53 −/− mice, regardless of TBI ( Supplementary Fig. 11 ). We then examined poly I:C-mediated cell death in p53 −/− mice. Similar to p53 +/+ mice, intraperitoneal injection of poly I:C induced cell death of crypt epithelial cells in p53 −/− mice ( Fig. 5e ). These results suggest that TLR3 on crypt cells is not activated in the absence of some p53-dependent event after irradiation. 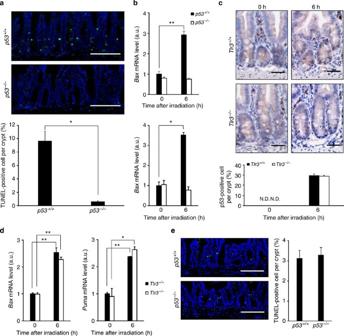Figure 5: TLR3-mediated crypt cell death after TBI depends on p53. (a) TUNEL-staining of small intestinal crypts ofp53+/+andp53−/−mice 6 h after TBI and isologous BMT. TUNEL-stained epithelium shows green fluorescence. Nuclei were stained with DAPI (blue). Scale bar: 100 μm. Lower panel shows numbers of TUNEL-positive cells.n=3; results are means±s.e.m. *P<0.05 (unpaired two-tailed Student’st-test). (b) Quantitative real-time PCR of mRNA encoding Bax and PUMA in the small intestines ofp53+/+andp53−/−mice.n=3; results are means±s.e.m. *P<0.05; **P<0.01 (unpaired two-tailed Student’st-test). (c) Immunohistochemical detection of p53 in the small intestinal crypts ofTlr3+/+andTlr3−/−mice 0 and 6 h after TBI and isologous BMT. Scale bar, 100 μm. Lower panel shows numbers of p53-positive cells.n=3; results are means±s.e.m. N.D., not detected. (d) Quantitative real-time PCR of mRNAs encoding Bax and PUMA in the small intestines ofTlr3+/+andTlr3−/−mice.n=3; results are means±s.e.m. *P<0.05; **P<0.01 (unpaired two-tailed Student’st-test). (e) TUNEL-staining of the small intestinal crypts ofp53+/+andp53−/−mice 6 h after poly I:C injection. TUNEL-stained epithelium shows green fluorescence. Nuclei were stained with DAPI (blue). Scale bar, 100 μm. The right-hand panel shows numbers of TUNEL-positive cells.n=3; results are means±s.e.m. Results are representative of three independent experiments. Figure 5: TLR3-mediated crypt cell death after TBI depends on p53. ( a ) TUNEL-staining of small intestinal crypts of p53 +/+ and p53 −/− mice 6 h after TBI and isologous BMT. TUNEL-stained epithelium shows green fluorescence. Nuclei were stained with DAPI (blue). Scale bar: 100 μm. Lower panel shows numbers of TUNEL-positive cells. n =3; results are means±s.e.m. * P <0.05 (unpaired two-tailed Student’s t -test). ( b ) Quantitative real-time PCR of mRNA encoding Bax and PUMA in the small intestines of p53 +/+ and p53 −/− mice. n =3; results are means±s.e.m. * P <0.05; ** P <0.01 (unpaired two-tailed Student’s t -test). ( c ) Immunohistochemical detection of p53 in the small intestinal crypts of Tlr3 +/+ and Tlr3 −/− mice 0 and 6 h after TBI and isologous BMT. Scale bar, 100 μm. Lower panel shows numbers of p53-positive cells. n =3; results are means±s.e.m. N.D., not detected. ( d ) Quantitative real-time PCR of mRNAs encoding Bax and PUMA in the small intestines of Tlr3 +/+ and Tlr3 −/− mice. n =3; results are means±s.e.m. * P <0.05; ** P <0.01 (unpaired two-tailed Student’s t -test). ( e ) TUNEL-staining of the small intestinal crypts of p53 +/+ and p53 −/− mice 6 h after poly I:C injection. TUNEL-stained epithelium shows green fluorescence. Nuclei were stained with DAPI (blue). Scale bar, 100 μm. The right-hand panel shows numbers of TUNEL-positive cells. n =3; results are means±s.e.m. Results are representative of three independent experiments. Full size image Gut microbiota is dispensable for crypt cell death after TBI We next examined which substances activated TLR3 to induce crypt cell death after TBI. The mammalian GI tract contains numerous species of microorganisms that constitute an intestinal microflora. Since TLR3 is known as a sensor for viral dsRNA, we studied crypt cell death in germ-free (GF) mice after TBI [9] , [10] , [15] . However, there were no differences between GF and specific pathogen-free (SPF) mice in terms of crypt cell death at 6 h or regeneration at 3 days after TBI, suggesting that the gut microbiota is not responsible for TLR3 activation following TBI ( Fig. 6a,b ). 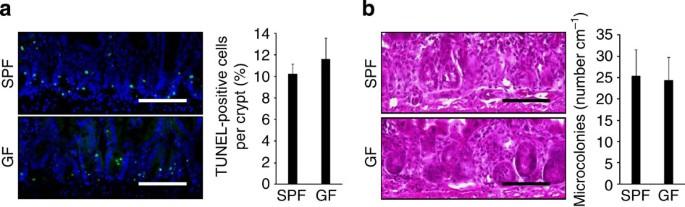Figure 6: The gut microbiota is not responsible for crypt cell death after TBI. (a) TUNEL-staining of small intestinal crypts of SPF and GF mice 6 h after TBI and BMT. TUNEL-stained epithelium shows green fluorescence. Nuclei were stained with DAPI (blue). Scale bar, 100 μm. The right-hand panel shows numbers of TUNEL-positive cells.n=3; results are means±s.e.m. (b) H&E staining of crypts of SPF and GF mice on day 3. Scale bar, 100 μm. The right-hand panel shows the numbers of microcolonies.n=3; results are means±s.e.m. Results are representative of two independent experiments. Figure 6: The gut microbiota is not responsible for crypt cell death after TBI. ( a ) TUNEL-staining of small intestinal crypts of SPF and GF mice 6 h after TBI and BMT. TUNEL-stained epithelium shows green fluorescence. Nuclei were stained with DAPI (blue). Scale bar, 100 μm. The right-hand panel shows numbers of TUNEL-positive cells. n =3; results are means±s.e.m. ( b ) H&E staining of crypts of SPF and GF mice on day 3. Scale bar, 100 μm. The right-hand panel shows the numbers of microcolonies. n =3; results are means±s.e.m. Results are representative of two independent experiments. Full size image Self-RNA induces TLR3-dependent crypt cell death In addition to the exogenous ligands derived from microbes, accumulating evidence has indicated that TLRs sense endogenous ligands released from injured tissues and induce inflammatory responses [28] . These endogenous ligands derived from ‘hosts’ are either cellular components or inducible gene products, such as intracellular constituents, extracellular matrix proteins and nucleic acids, and exacerbate tissue damage via TLR activation. Therefore, we assumed that an endogenous molecule might be involved in TLR3-mediated crypt cell death after TBI. We first investigated whether small intestine homogenates after 10-Gy TBI could stimulate interferon-stimulated response element (ISRE) reporter activity through TLR3. Interestingly, the small intestinal homogenate significantly stimulated ISRE reporter activity in HEK293 cells when transiently transfected with an expression plasmid encoding TLR3 ( Fig. 7a ). Moreover, treatment with RNase, but not with proteinase or DNase, diminished the capability of the small intestinal homogenate to stimulate ISRE reporter activity through TLR3. Thus, RNA in the small intestinal homogenate was supposed to stimulate TLR3. We then examined whether irradiation damage causes a leakage of cellular RNA using an in vitro crypt culture system. We cultured small intestinal crypts from p53 +/+ and p53 −/− mice and examined the morphological changes and viability of the organoids after γ-irradiation. Following γ-irradiation, crypt domains disappeared from p53 +/+ organoids, but not from p53 −/− organoids ( Supplementary Fig. 12 ). An MTT assay showed that γ-irradiation significantly reduced the cell viability of p53 +/+ organoids, but not of p53 −/− organoids. Thus, crypt cell death occurred by γ-irradiation in vitro in a p53-dependent manner. We then analysed total RNA from the culture supernatant using an Agilent 2100 bioanalyzer, which is commonly used for measuring the quantity and size distribution of nucleic acids. Interestingly, RNA molecules varying from about 25 to 1,000 nucleotides (nt) in length were detected in the culture supernatants of p53 +/+ organoids, but not in those of p53 −/− organoids, after γ-irradiation ( Fig. 7b ). Furthermore, we compared radiation-induced cell death of crypt–villus organoids between Tlr3 +/+ and Tlr3 −/− mice. Compared with Tlr3 +/+ organoids, the disappearance of crypt domains after irradiation was apparently milder in Tlr3 −/− organoids ( Fig. 7c ). In addition, the cell viability of Tlr3 −/− organoids was significantly higher than that of Tlr3 +/+ organoids. Interestingly, when the organoids were incubated with RNase, atrophy of Tlr3 +/+ organoids was ameliorated and the viability increased to the levels comparable to that of Tlr3 −/− organoids. Taken together, these findings suggest that endogenous RNA originating from crypt cells that underwent p53-dependent cell death after γ-irradiation may induce extensive cell death via TLR3. 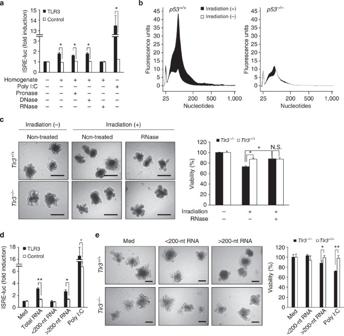Figure 7: Cellular RNA leaks from irradiated crypt cells in a p53-dependent manner and induces TLR3-mediated crypt cell death. (a) HEK293 cells transiently transfected with a human TLR3 expression vector together with ISRE-luciferase reporter plasmid (HEK293-hTLR3) were incubated with homogenate from irradiated small intestine or homogenate treated with pronase, DNase or RNase. Reporter activity was measured in triplicate. Results are means±s.e.m. *P<0.05 (unpaired two-tailed Student’st-test). (b) Quantification and size distribution of total RNA in the culture supernatants of crypt–villus organoids ofp53+/+andp53−/−mice on day 1 after irradiation. (c) Representative images of crypt–villus organoids ofTlr3+/+andTlr3−/−mice on day 1 after irradiation. Crypts were treated without or with RNase. Scale bar, 200 μm. The right-hand panel shows the viability. Viability was measured in triplicate. Results are means±s.e.m. N.S., not significant. *P<0.05 (unpaired two-tailed Student’st-test). (d) HEK293-hTLR3 cells were incubated with medium alone (Med), purified RNA or poly I:C for 12 h. Reporter activity was measured in triplicate. Results are means±s.e.m. *P<0.05; **P<0.01 (unpaired two-tailed Student’st-test). (e) Representative images ofin vitrocultured crypts ofTlr3+/+andTlr3−/−mice (left) and the viability (right) on day 2 after treatment with Med or purified RNA. Scale bar, 200 μm. Viability was measured in triplicate. Results are means±s.e.m. *P<0.05; **P<0.01 (unpaired two-tailed Student’st-test). Results are representative of three independent experiments. Figure 7: Cellular RNA leaks from irradiated crypt cells in a p53-dependent manner and induces TLR3-mediated crypt cell death. ( a ) HEK293 cells transiently transfected with a human TLR3 expression vector together with ISRE-luciferase reporter plasmid (HEK293-hTLR3) were incubated with homogenate from irradiated small intestine or homogenate treated with pronase, DNase or RNase. Reporter activity was measured in triplicate. Results are means±s.e.m. * P <0.05 (unpaired two-tailed Student’s t -test). ( b ) Quantification and size distribution of total RNA in the culture supernatants of crypt–villus organoids of p53 +/+ and p53 − / − mice on day 1 after irradiation. ( c ) Representative images of crypt–villus organoids of Tlr3 +/+ and Tlr3 −/− mice on day 1 after irradiation. Crypts were treated without or with RNase. Scale bar, 200 μm. The right-hand panel shows the viability. Viability was measured in triplicate. Results are means±s.e.m. N.S., not significant. * P <0.05 (unpaired two-tailed Student’s t -test). ( d ) HEK293-hTLR3 cells were incubated with medium alone (Med), purified RNA or poly I:C for 12 h. Reporter activity was measured in triplicate. Results are means±s.e.m. * P <0.05; ** P <0.01 (unpaired two-tailed Student’s t -test). ( e ) Representative images of in vitro cultured crypts of Tlr3 +/+ and Tlr3 −/− mice (left) and the viability (right) on day 2 after treatment with Med or purified RNA. Scale bar, 200 μm. Viability was measured in triplicate. Results are means±s.e.m. * P <0.05; ** P <0.01 (unpaired two-tailed Student’s t -test). Results are representative of three independent experiments. Full size image We next isolated RNAs from the small intestine after TBI and examined whether they could stimulate ISRE reporter activity through TLR3. Total RNA derived from irradiated small intestine significantly upregulated ISRE reporter activity in a TLR3-dependent manner ( Fig. 7d ). As shown in Fig. 7b , small RNAs less than 200-nt in length were detected in the culture supernatants of p53 +/+ organoids after γ-irradiation. Recently, a small interfering RNA (siRNA) was shown to suppress angiogenesis via TLR3 (ref. 29 ). Therefore, we supposed that host-derived small non-coding RNAs, such as microRNAs, are involved in TLR3-mediated crypt cell death after TBI. However, small RNAs (<200-nt) did not stimulate ISRE reporter activity through TLR3 ( Fig. 7d and Supplementary Fig. 13a–c ). Contrary to our expectations, large RNAs (>200-nt) significantly stimulated ISRE reporter activity through TLR3. We next examined whether large RNAs induced crypt cell death in vitro . Large RNAs, but not small RNAs, induced breakdown of crypt–villus organoids from Tlr3 +/+ but not Tlr3 −/− mice ( Fig. 7e ). Cell viability was significantly decreased in Tlr3 +/+ organoids but not in Tlr3 −/− organoids after treatment with large RNAs. Thus, large RNAs derived from irradiated small intestinal cells may induce crypt cell death via TLR3. TLR3/dsRNA complex inhibitor protects mice from GIS The aforementioned results raise the possibility that endogenous RNA induces TLR3-dependent crypt cell death in GIS. To elucidate the in vivo mechanism, we used ( R )-2-(3-chloro-6-fluorobenzo[b]thiophene-2-carboxamido)-3-phenylpropanoic acid, a competitive inhibitor of dsRNA binding to TLR3 (ref. 30 ). We also confirmed that this small molecule suppressed upregulation of mRNA encoding IL-12p40 in CD8α + splenic dendritic cells after poly I:C stimulation ( Supplementary Fig. 14 ), which is completely dependent on TLR3 (ref. 31 ). Treatment of mice with the TLR3 inhibitor before TBI significantly improved their survival and ameliorated diarrhea and weight loss ( Fig. 8a–c ). Moreover, the TLR3 inhibitor pretreatment significantly reduced crypt cell death and increased microcolonies 6 h and 3 days after TBI, respectively ( Fig. 8d,e ). Finally, inhibitor treatment resulted in significant improvements in survival and GIS symptoms, even when administered after TBI ( Fig. 9a–c ). Thus, inhibition of TLR3/dsRNA binding effectively reduced crypt cell death and protected mice from GIS. 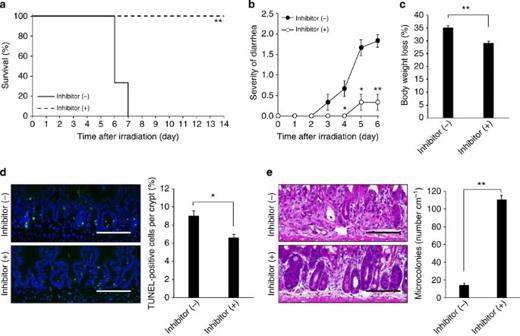Figure 8: Blockade of TLR3 binding to RNA ameliorates radiation-induced GIS. (a) Kaplan–Meier survival analyses of mice treated with TLR3/dsRNA complex inhibitor before TBI and isologous BMT.n=6; **P<0.01 (log-rank test). (b,c) Severity of diarrhea (b) and body weight loss (c) of non-treated and TLR3/dsRNA complex inhibitor-pretreated mice.n=6; results are means±s.e.m. *P<0.05; **P<0.01 (unpaired two-tailed Student’st-test). (d) TUNEL-staining of the small intestinal crypts of non-treated and TLR3/dsRNA complex inhibitor-pretreated mice at 6 h. TUNEL-stained epithelium shows green fluorescence. Nuclei were stained with DAPI (blue). Scale bar, 100 μm. The right-hand panel shows numbers of TUNEL-positive cells.n=5; results are means±s.e.m. *P<0.05 (unpaired two-tailed Student’st-test). (e) H&E staining of the small intestinal crypts of non-treated and TLR3/dsRNA complex inhibitor-pretreated mice on day 3. Scale bar: 100 μm. Asterisks denote microcolonies. Right panel shows the numbers of microcolonies.n=5; results are means±s.e.m. **P<0.01 (unpaired two-tailed Student’st-test). Results are representative of three independent experiments. Figure 8: Blockade of TLR3 binding to RNA ameliorates radiation-induced GIS. ( a ) Kaplan–Meier survival analyses of mice treated with TLR3/dsRNA complex inhibitor before TBI and isologous BMT. n =6; ** P <0.01 (log-rank test). ( b , c ) Severity of diarrhea ( b ) and body weight loss ( c ) of non-treated and TLR3/dsRNA complex inhibitor-pretreated mice. n =6; results are means±s.e.m. * P <0.05; ** P <0.01 (unpaired two-tailed Student’s t -test). ( d ) TUNEL-staining of the small intestinal crypts of non-treated and TLR3/dsRNA complex inhibitor-pretreated mice at 6 h. TUNEL-stained epithelium shows green fluorescence. Nuclei were stained with DAPI (blue). Scale bar, 100 μm. The right-hand panel shows numbers of TUNEL-positive cells. n =5; results are means±s.e.m. * P <0.05 (unpaired two-tailed Student’s t -test). ( e ) H&E staining of the small intestinal crypts of non-treated and TLR3/dsRNA complex inhibitor-pretreated mice on day 3. Scale bar: 100 μm. Asterisks denote microcolonies. Right panel shows the numbers of microcolonies. n =5; results are means±s.e.m. ** P <0.01 (unpaired two-tailed Student’s t -test). Results are representative of three independent experiments. 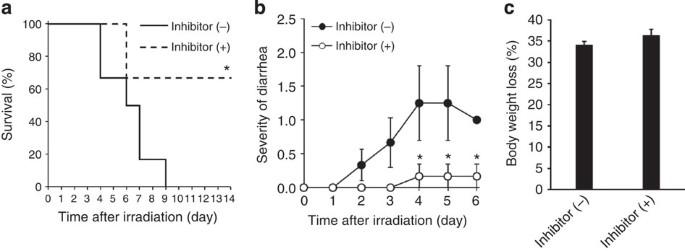Figure 9: Post-treatment with TLR3/dsRNA complex inhibitor ameliorates radiation-induced GIS. (a) Kaplan–Meier survival analyses of mice treated with TLR3/dsRNA complex inhibitor after TBI and isologous BMT.n=6; *P<0.05 (log-rank test). (b,c) Severity of diarrhea (b) and body weight loss (c) of non-treated and TLR3/dsRNA complex inhibitor-post-treated mice.n=4–6; results are means±s.e.m. *P<0.05 (unpaired two-tailed Student’st-test). Results are representative of two independent experiments. Full size image Figure 9: Post-treatment with TLR3/dsRNA complex inhibitor ameliorates radiation-induced GIS. ( a ) Kaplan–Meier survival analyses of mice treated with TLR3/dsRNA complex inhibitor after TBI and isologous BMT. n =6; * P <0.05 (log-rank test). ( b , c ) Severity of diarrhea ( b ) and body weight loss ( c ) of non-treated and TLR3/dsRNA complex inhibitor-post-treated mice. n =4–6; results are means±s.e.m. * P <0.05 (unpaired two-tailed Student’s t -test). Results are representative of two independent experiments. Full size image Crypts are tubular glands found in the epithelial lining of the small intestine [18] , [32] . The basal portion of crypts contains multipotent stem cells, which continuously divide and supply the transit-amplifying progenitors for all epithelial cell lineages [32] , [33] . After terminal differentiation, newly formed functional epithelial cells migrate up the adjacent villus and eventually exfoliate from the apical tip. The transit time of epithelial cells from the basal area of the crypt to the tip of villus is about 3 days. Thus, the epithelium in small intestine is one of the most rapidly renewing tissues, and epithelial cells, especially stem cells in crypts, are very sensitive to radiation injury. Recent studies have reported that stimulation of TLR2, 4, 5 or 9 by ligand administration enhances anti-apoptotic activities, leading to amelioration of radiation-induced crypt cell death [11] , [12] , [13] , [14] , [34] . However, the therapeutic application of TLR agonists seems to be difficult, because their administration can also enhance inflammation in damaged tissues after exposure to irradiation. In the present study, we investigated the radiation susceptibilities of TLR-knockout mice to evaluate the impact of TLR deficiency on GIS. A recent study has suggested that Myd88 − / − mice showed marked resistance to GIS [35] . However, our study revealed that there was no attenuation of GIS in mice deficient in TLR2, 4, 5, 7 and 9. Thus, each TLR has a limited role in the pathogenesis of GIS in the absence of artificial administration of TLR ligands. Interestingly, we identified that mice deficient in TLR3 showed significant resistance to GIS. When exposed to 10-Gy TBI, mice acutely die of HPS or GIS [16] . Although HPS was induced in Tlr3 −/− mice to a similar extent to that in Tlr3 +/+ mice, GIS symptoms, such as diarrhea and body weight loss, were apparently milder in Tlr3 −/− mice. Atrophy and disappearance of crypts occurred in Tlr3 +/+ mice on day 3 after TBI owing to marked cell death of crypt epithelial cells, leading to destruction of villous epithelium in the small intestine at day 5. There were no differences in cell death of villous epithelium or accumulation of inflammatory cells between Tlr3 +/+ and Tlr3 −/− mice. In contrast to Tlr3 +/+ mice, crypt cell death was significantly milder in Tlr3 −/− mice 6 h after TBI and the crypt structure was still retained in Tlr3 −/− mice at day 3. As cell proliferation was active in the crypts of Tlr3 −/− mice at day 3, the surviving crypts, which retain intestinal stem cells, might promote the re-epithelization of small intestinal villi, preventing death from GIS. The present study showed that TLR3-mediated crypt cell death after irradiation is dependent on TRIF and RIP1. In addition, we observed TLR3-dependent activation of caspase-3 in crypt cells after irradiation or poly I:C administration. Thus, apoptosis is the cause of crypt cell death induced by TLR3/TRIF/RIP1 signalling. Importantly, the RIP1 pathway downstream of TLR3 was reported to activate NF-κB simultaneously with apoptosis induction [36] . Although administration of other TLR ligands exerted protective effects on crypt cells against irradiation by inducing anti-apoptotic genes via NF-κB [11] , [12] , [13] , TLR3/TRIF/RIP1 signalling induced apoptosis. Previous studies have suggested that RIP1-mediated cell death was not affected by NF-κB activation [21] , [37] , [38] , [39] . Therefore, TLR3/TRIF/RIP1 signalling may promote cell death but not protective functions in crypts after TBI. It is generally accepted that ionizing radiation-induced cell death is regulated via a p53-dependent machinery in the GI tract [4] , [40] . Although crypt cell death was milder, neither p53 accumulation in crypt cells nor the subsequent induction of pro-apoptotic genes such as Bax and PUMA were impaired in Tlr3 −/− mice after TBI. On the other hand, TLR3-mediated crypt cell death by poly I:C was normally induced in p53 −/− mice. As crypt cell death was almost completely diminished in p53 −/− mice after TBI, TLR3-mediated crypt cell death seemed to be attributable to a p53-dependent response. TLR3 was originally identified as a sensor for viral or synthetic dsRNA but not homopolymer single-stranded (ss) RNA [9] , [10] , [15] . Furthermore, previous studies have revealed that GF mice are markedly resistant to radiation-induced GIS. Compared with conventionally raised mice, GF mice survived longer owing to the alleviation of enteritis [41] . Therefore, we anticipated that substances derived from commensal flora activate TLR3 to induce crypt cell death after TBI. Unexpectedly, we observed no difference in crypt cell death between GF and SPF mice after TBI. Thus, the resident flora is not involved in TLR3-mediated crypt cell death after TBI. GF mice may avoid gastroenteritis due to secondary infection and show resistance to GIS. In addition to viral dsRNA, recent reports have shown that host-derived RNAs activate TLR3 (refs 42 , 43 , 44 , 45 ). Interestingly, RNA leaked from crypt–villus organoids after γ-irradiation in a p53-dependent manner. Although the leaking RNAs were predominantly small RNAs of less than 200-nt length, large RNAs were also detected in the culture supernatants after γ-irradiation. A recent report showed that a siRNA suppresses neovascularization in mice via sequence-independent activation of cell surface TLR3 (ref. 29 ). Unexpectedly, small RNAs derived from the irradiated small intestine could not activate TLR3. In contrast, large RNAs induced TLR3-mediated ISRE reporter activation and cell death in crypt–villus organoids in a TLR3-dependent manner. According to a report by Liu et al. [46] , TLR3 binds as dimers to dsRNA and requires a length of at least 40–50 base pairs for binding to a single dsRNA. Therefore, there may also be a minimum length for mammalian RNAs to bind TLR3. However, although large RNAs could activate TLR3, such RNAs are typically regarded as ssRNAs. Importantly, a recent report showed that poliovirus-derived ssRNA segments harbouring stem structures with bulge/internal loops can activate TLR3 (ref. 47 ). This report also suggested that a relatively longer stem structure with a bulge and internal loops is required for TLR3 activation. Thus, we assume that mammalian ssRNAs >200-nt in length may also form long double-strand-like structures potentially capable of activating TLR3. However, these ssRNAs with bulge/internal loops seem to make up only a small portion of the >200-nt ssRNAs isolated from irradiated small intestines. In contrast, poly I:C is a synthetic analogue of dsRNA that consists mainly of dsRNAs of sufficient length [48] . Therefore, the less stimulatory effect of large RNAs compared with poly I:C at the same concentration was likely due to its lower content of long dsRNAs. Additionally, previous studies have reported that self-derived nucleic acids form complexes with endogenous proteins in some inflammatory and autoimmune diseases, which in turn promote inflammation by activating TLRs [28] . Further studies will be needed to clarify the type, structure, potential interaction with other molecules, stability and mode of association with TLR3 of large RNAs derived from radiation-damaged crypt cells. In addition to radiation exposure in nuclear accidents, extensive abdominal irradiation used in treatments for metastases of whole-body lymph nodes and peritoneal dissemination of ovarian cancers also results in serious side effects similar to GIS [33] . To date, amifostine is the only radioprotectant approved for use in humans [49] . Amifostine decreases radiation-induced DNA damage primarily by blocking the formation of free radicals resulting from ionization of water and other molecules in the cytoplasm [50] . Regardless of the clinical and experimental evidence supporting the activity of amifostine in the prevention of radiation toxicity toward the GI tract [50] , the drug is currently being used in patients undergoing radiation therapy solely for reducing or preventing acute or late xerostomia, because of the many negative effects such as hypotension, nausea, vomiting and allergic reactions [49] . p53 has been suggested as a primary causal factor of radiation-induced crypt cell death. However, previous studies have shown that p53 deficiency does not protect mice from GIS [8] , [40] . In p53 − / − crypt cells, p53-mediated cell death as well as DNA repair functions are abolished after irradiation. Eventually, p53 − / − cells with DNA damage are killed by p53-independent reproductive or mitotic death [8] , [40] . Therefore, drugs to treat GIS should not compromise the DNA-repair activity of p53. Thus, although reducing radiation-induced cell death would be desirable for the prevention of GIS, no effective clinical treatment is yet available. The present study clearly showed that self-RNAs derived from the damaged small intestine after TBI induce extensive crypt cell death via TLR3, leading to lethal disturbance of the GI tract. While p53 serves as an initial trigger for GIS, TLR3 is critical for exacerbation of GIS ( Fig. 10 ). We would strongly emphasize that TLR3 is a preferable therapeutic target for GIS, not only because TLR3 is directly involved in the pathogenesis, but also because blockade of TLR3 does not affect p53-mediated DNA repair functions. In this study, we showed that blockade of TLR3 signalling by an inhibitor of TLR3/dsRNA complex formation and by Nec-1 effectively ameliorated GIS. We propose that the TLR3/dsRNA complex inhibitor is particularly effective for the treatment of GIS. This inhibitor exerted a protective effect against GIS with fewer injections compared with Nec-1. As the Nec-1 target RIP1 is a downstream molecule in the TLR3 signalling pathway, the inhibitory effect of Nec-1 would be less than that of the inhibitor of TLR3/dsRNA complex formation, which blocks signalling at the receptor level. It is also important to note that the TLR3/dsRNA complex inhibitor is highly protective against GIS, even when administered after radiation exposure. Future studies based on these findings will provide therapeutic clinical options for the prevention of GIS in radiation therapy, as well as for the treatment of victims of nuclear accidents. 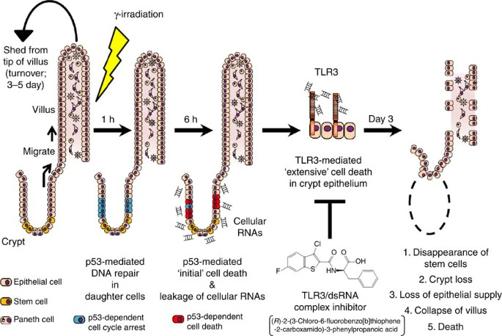Figure 10: Whole pathological mechanism of GIS. When ionizing γ-radiation damages DNA of intestinal crypt cells, p53 induces cell cycle arrest for DNA repair. If the DNA damage is irreparable, p53 initiates cell death. Cellular RNA released from the cells, which underwent p53-mediated cell death after γ-irradiation, induces extensive crypt cell death via TLR3, leading to a deficient supply of intestinal epithelial cells, destruction of villous epithelium and death from GIS. Figure 10: Whole pathological mechanism of GIS. When ionizing γ-radiation damages DNA of intestinal crypt cells, p53 induces cell cycle arrest for DNA repair. If the DNA damage is irreparable, p53 initiates cell death. Cellular RNA released from the cells, which underwent p53-mediated cell death after γ-irradiation, induces extensive crypt cell death via TLR3, leading to a deficient supply of intestinal epithelial cells, destruction of villous epithelium and death from GIS. Full size image Mice Wild-type BALB/c mice (female, 8–12 weeks old) kept under SPF or GF conditions were purchased from CLEA Japan. Tlr2 − / − , Tlr3 − / − , Tlr4 − / − , Tlr5 − / − , Tlr7 − / − , Tlr9 − / − , Trif − / − and Irf3 − / − mice [20] , [51] , [52] , [53] , [54] , [55] , [56] were backcrossed onto a BALB/c background for more than eight generations. Ifnar −/− mice (BALB/c) [57] and p53 −/− mice (BALB/c) [58] were generated by breeding heterozygote-deficient mice, which were kindly donated by S. Miyatake and N. Mori, respectively. Mice were housed in standard cages in a temperature-controlled room under a 12-h light/dark cycle in an SPF environment in the Animal Resource Center for Infectious Diseases at Osaka University. They were granted free access to standard laboratory mouse chow and drinking water. GF mice were maintained in vinyl isolators at the experimental animal facility of the Institute of Medical Science at the University of Tokyo. They were maintained under 12-h light/dark cycle and provided with autoclaved diet and sterilized water ad libitum . All animal experiments were carried out with the approval of the Animal Research Committee of the Research Institute for Microbial Diseases at Osaka University and Animal Care and Use Committees of The University of Tokyo. Poly I:C treatment Poly I:C (Poly I:C-HMW, Invivogen) was diluted in pathogen-free PBS without using a transfecting reagent or liposomal vehicle. Poly I:C was injected into mice intraperitoneally. Nec-1 treatment Nec-1 (Sigma-Aldrich) was dissolved in DMSO and diluted in pathogen-free PBS. Nec-1 was administered to mice by intraperitoneal injection, several times, to achieve a significant protective effect against GIS. TLR3/dsRNA complex inhibitor treatment The TLR3/dsRNA complex inhibitor (( R )-2-(3-Chloro-6-fluorobenzo [b] thiophene-2 -carboxamido)-3-phenylpropanoic acid, Calbiochem) was dissolved in DMSO and diluted in pathogen-free PBS. The inhibitor was intraperitoneally injected into mice several times as described below. Radiation treatment Mice (female, 8–12 weeks old) were exposed to 10 Gy of TBI at a dose rate of 88 cGy min − 1 using a 137 Cs irradiator (Gammacell 40 Exactor; MDS Nordion). In some experiments, mice were injected with poly I:C (20 mg per kg body weight) at 1 h before irradiation. Nec-1 (125 mg per kg body weight) was administered 1 h before and 2, 24, 48 and 72 h after irradiation. The TLR3/dsRNA complex inhibitor (1 mg per mouse) was administered 1 h before or 1 h after irradiation. Subsequently, mice were injected with the inhibitor at 24 and 48 h. Unless otherwise noted, mice subsequently received a single intravenous injection of 1 × 10 7 BM cells obtained from strain-, sex- and genotype-matched donor mice. Mice were given 1,000 U ml − 1 polymixin B and 1 mg ml − 1 neomycin in drinking water after irradiation. The clinical severity of GIS was evaluated by observing body weight loss and diarrhea. The latter was scored daily by checking the evidence of diarrhea on the fur in the anal region as follows: 0, no evidence; 1, light brown stool; 2, tar-like black stool. Blood and BM leukocyte counts Blood was collected from the retro-orbital vein at 0 and 5 days after irradiation. Erythrocytes were eliminated by treating blood with red blood cell lysing buffer (Sigma-Aldrich). Thereafter, cells were suspended in PBS and an aliquot was mixed with Turk’s solution for leukocyte counting using a hemocytometer. BM cells were harvested from femurs by flushing with Hank’s balanced salt solution using a 28-gauge needle and syringe at 0 and 5 days after irradiation. Erythrocyte lysis and leukocyte counting were performed as described above. Histological analysis At 0, 6, 72 and 120 h after radiation or poly I:C treatment, jejunal tissues were excised from small intestine 4 cm below the gastroduodenal junction, flushed with PBS, fixed in 10% formalin overnight and embedded in paraffin. Five-micrometre sections were stained with hematoxylin and eosin (H&E) and observed under a light microscope using BZ-II Image Analysis Application (BZ-9000, Keyence). Crypt survival was evaluated at 3 days after irradiation by a modification of microcolony assay [17] . Briefly, the numbers of regenerating crypts in jejunal sections were counted based on histological appearance. Regenerating crypts were defined as those containing ≥10 adjacent chromophilic non-Paneth cells and at least one Paneth cell. Tibias were collected at 0 and 5 days after irradiation, fixed in 70% ethanol for 3 days, embedded in methyl methacrylate resin and stained with H&E. Cell death in the small intestine was evaluated by TUNEL-staining. Paraffin sections of small intestine were treated with reagents supplied in the in situ Cell Death Detection Kit, Fluorescein (Roche Diagnostics). Samples were mounted in ProLong Gold Antifade Reagent with DAPI (Invitrogen) and observed under a fluorescence microscope using BZ-II Image Analysis Application. At least 50 crypts were counted to calculate the numbers of TUNEL-positive cells per crypt. Immunohistochemical analysis To label proliferating S-phase cells in the small intestine, mice were intraperitoneally injected with BrdU (5-bromo-2′-deoxyuridine; 50 mg kg − 1 body weight) at 1 h before being killed. Paraffin sections of small intestine were prepared as described above. Endogenous peroxidase activity was quenched with 3% hydroperoxide for 10 min. Sections were treated with 2N HCl for 30 min, blocked with 10% goat serum in PBS for 30 min and stained with mouse anti-BrdU antibody (100 × , Ab-3, Lab Vision Corporation) overnight at 4 °C. Sections were washed and then were incubated with biotin-conjugated goat anti-mouse IgG (1,500 × , Kirkegaard & Perry Laboratories) for 1 h at 37 °C, followed by incubation with streptavidin-conjugated horseradish peroxidase (Thermo Fisher Scientific) for 30 min at room temperature. Sections were visualized with 3, 3′-diaminobenzidine and hydroperoxide and counterstained with hematoxylin. The numbers of BrdU-positive cells were counted in at least 50 crypts. To detect accumulation of p53 protein, sections were treated with mouse anti-p53 antibody ( × 100, PAb 240, Abcam) overnight at 4 °C, following antigen retrieval by heating in citrate buffer (pH 6.0) for 15 min at 121 °C. Detection of primary antibody and visualization were performed as described above. Active form caspase-3 was detected using rabbit anti-cleaved caspase-3 antibody (100 × , 5A1E, Cell Signaling Technology) as described above. Bound primary antibody was detected using biotin-conjugated goat anti-rabbit IgG (1,500 × , Kirkegaard & Perry Laboratories) for 1 h at 37 °C and visualization was performed as described above. The numbers of positive cells were counted in at least 50 crypts. RT-PCR and quantitative real-time PCR Villus, crypt and lamina propria cells were prepared from the small intestine according to the methods described by Fujimoto et al. [59] and Sato et al. [18] . Briefly, tissue fragments of small intestine were incubated with 2 mM EDTA in PBS for 30 min on ice. After removal of EDTA, repeated vigorous shaking of the sample with cold PBS and centrifugation yielded supernatant fractions enriched in villus and crypt. For isolation of lamina propria cells, small intestinal segments were treated with PBS containing 10% FCS and 10 mM EDTA for 30 min at 37 °C to remove epithelial cells, followed by extensive washing with fresh PBS. Small intestinal segments were digested with 0.425 mg ml −1 Liberase T-flex (Roche) and 100 μg ml −1 DNase I (Roche) in RPMI 1640 supplemented with 10% fetal calf serum with continuous stirring at 37 °C for 60 min. The suspended cells were subjected to density-gradient centrifugation in 40 and 75% (vol/vol) Percoll. Cells collected from the interface were washed and used as lamina propria cells. Total RNA was isolated using Trizol reagent (Invitrogen) according to the manufacturer’s instructions. Subsequently, RQ1 RNase-free DNase (Promega) was added to the total RNA sample, followed by incubation for 45 min at 37 °C. After purification by phenol–chloroform extraction, total RNA was precipitated with ethanol and then re-suspended in double-distilled water. Two micrograms of total RNA was reverse-transcribed using SuperScript III First-Strand Synthesis SuperMix (Invitrogen) according to the manufacturer’s instructions with random hexamers as primers. The sequences of primers used for PCR were as follows: Tlr3 ; 5′-CAGTTCAGAAAGAACGG-3′ (forward) and 5′-AGCCTTATACCATAAAAG C-3′ (reverse), actin ; 5′-GACATGGAGAAGATCTGGCACCACA-3′ (forward) and 5′-ATCTCCTGCTCGAAGTCTAGAGCAA-3′ (reverse). The primer pairs and Taq polymerase (Takara Shuzo) were used for PCR under the following conditions: 5 min at 94 °C; 30 cycles of 30 s at 97 °C, 30 s at 57 °C, 30 s at 72 °C, and 7 min at 72 °C. The products were then separated by agarose gel electrophoresis. Quantitative real-time PCR was carried out in a final volume of 25 μl containing cDNA, Real-time PCR Master Mix (Toyobo), and primers specific for 18S rRNA (Applied Biosystems) as an internal control or primers specific for Tlr3, Bax or Puma (Applied Biosystems), using an ABI Prism 7700 sequence detection system (Applied Biosystems). After incubation at 95 °C for 10 min, products were amplified under the following conditions: 35 cycles of 15 s at 95 °C, 60 s at 60 °C and 120 s at 50 °C. Preparation of small and large RNA fractions Total RNA was isolated as described above and further divided into small (<200-nt) and large RNA fractions (>200-nt) using an miRNeasy Mini Kit and an RNeasy MinElute Cleanup Kit (Qiagen). The sizes of separated RNA were confirmed using an Agilent 2100 Bioanalyzer with an Agilent RNA 6000 Pico Kit (Agilent Technologies) ( Supplementary Fig. 13 ). In vitro crypt culture Small intestinal crypts were isolated according to the method as described above. Crypts were directly mounted in Matrigel (BD Biosciences), followed by seeding of a 48-well flat-bottom plate with 100 μl of Matrigel containing 200 crypts. Each well was overlaid with Advanced DMEM/F12 (Invitrogen) containing 2% fetal calf serum, 100 U ml − 1 penicillin, 100 μg ml − 1 streptomycin, 10 mM HEPES, Glutamax (Invitrogen), 1 × N2 (Invitrogen), 1 × B27 (Invitrogen), 1 μM N-acetylcysteine (Nacalai Tesque), 10 μM Y-27632 (Stemgent) and growth factors (50 ng ml − 1 epidermal growth factor, 100 ng ml − 1 noggin and 1 μg ml − 1 R-spondin-1) (all from R&D Systems). Medium was added every other day and the entire medium was replaced after 4 days of culture. Y-27632 was then withdrawn and not included in subsequent culture maintenance. At 5–6 days of culture, crypts were treated with either 100 μg ml − 1 purified RNA or poly I:C complexed with Lipofectamine 2000 reagent, or exposed to 10 Gy of irradiation. For enzymatic digestion assays, crypts were incubated with 5 μg ml − 1 DNase-free RNase (Roche Diagnostics). The images of cultured crypts were taken using a light microscope with the BZ-II Image Analysis Application. To evaluate the killing effects of irradiation or RNA on cultured crypt, cell viability was measured by MTT (3-(4,5-dimethyl-2-thiazolyl)-2,5-diphenyltetrazolium bromide) assay using an MTT cell count kit (Nacalai Tesque). Crypts were cultured with 500 μg ml − 1 MTT for 1 h and recovered from Matrigel using Cell Recovery Solution (BD Bioscience). After solubilizing formazans precipitated in crypts, the absorbance at 570 nm was measured. The percentage of crypt cell viability was calculated via the following formula; % cell viability=(value of treated crypt cells/value of untreated crypt cells) × 100. For whole-mount analysis, cultured crypts were directly fixed with 4% paraformaldehyde after recovering from the Matrigel and stained using the in situ Cell Death Detection Kit, Fluorescein. Nuclei were stained with 10 μg ml − 1 DAPI (4′,6′-diamidino-2-phenylindole). Images were acquired using a fluorescence microscope with the BZ-II Image Analysis Application. For quantification of RNA in the culture supernatant, SUPERase-In RNase Inhibitor (Ambion) was added at a concentration of 0.5 U μl − 1 . At 1 day after irradiation, the supernatant was collected and subjected to RNA extraction using Trizol LS reagent (Invitrogen) according to the manufacturer’s instructions. Quantification of purified RNA was performed using an Agilent 2100 Bioanalyzer with Agilent RNA 6000 Pico Kit. Preparation of intestinal homogenates Small intestine was dissected at 6 h following 10 Gy of irradiation, thoroughly washed with sterilized PBS, homogenized with DMEM and centrifuged at 15,000 g for 3 min. The supernatant was used as intestinal homogenate. For enzymatic digestion assays, the intestinal homogenate was incubated with 10 U ml − 1 pronase, 10 U ml − 1 RNase-free DNase or 5 μg ml − 1 DNase-free RNase (all from Roche Diagnostics) at 37 °C for 1 h. Reporter assay HEK293 cells (ATCC) were cultured in DMEM supplemented with 10% fetal calf serum at 37 °C in a 5% CO 2 incubator. HEK293 cells were transiently transfected with ISRE-luciferase reporter plasmid together with an expression vector plasmid pUNO-hTLR3 or an empty control vector pUNO-mcs (Invivogen) using Lipofectamine 2000 reagent. After 12 h, cells were seeded into 96-well flat-bottom plates at 5 × 10 4 cells per well. Thereafter, cells were incubated with 20 μg ml − 1 purified RNA or 0.5 μg ml − 1 poly I:C complexed with Lipofectamine 2000 reagent, or intestinal homogenate. After 12 h of cultivation, cells were harvested and lysed with passive lysis buffer (Promega) and their luciferase activities were measured using a Dual-Luciferase Reporter Assay System (Promega). TK promoter-driven Renilla luciferase plasmid was used as an internal control. CD8α + splenic dendritic cell culture CD8α + dendritic cells were purified from the spleen of wild-type mice (female, 8–12 weeks old) by magnetic sorting using the CD8 + Dendritic Cell Isolation kit (Miltenyi Biotec). The purity of the sorted DCs was routinely >95%. CD8α + dendritic cells were seeded into 96-well U-bottom plates at 5 × 10 4 cells per well and cultured in 200 μl of RPMI1640 containing 10% fetal calf serum at 37 °C in a 5% CO 2 incubator. Cells were pretreated with 100 μM TLR3/dsRNA complex inhibitor for 1 h before stimulation with 10 μg ml − 1 poly I:C. After 12 h of incubation, the expression levels of mRNAs encoding IL-12p40, IFN-α4 and IFN-β were measured by quantitative real-time PCR. Statistical analysis Statistical significance was evaluated using unpaired two-tailed Student’s t -tests. Kaplan–Meier plots and log-rank tests were used to assess the differences in survival between the groups after irradiation. P values less than 0.05 were considered to be statistically significant. How to cite this article: Takemura, N. et al. Blockade of TLR3 protects mice from lethal radiation-induced gastrointestinal syndrome. Nat. Commun. 5:3492 doi: 10.1038/ncomms4492 (2014).